The clathrin adaptor AP-1 complex and Arf1 regulate planar cell polarityin vivo A key step in generating planar cell polarity (PCP) is the formation of restricted junctional domains containing Frizzled/Dishevelled/Diego (Fz/Dsh/Dgo) or Van Gogh/Prickle (Vang/Pk) complexes within the same cell, stabilized via Flamingo (Fmi) across cell membranes. Although models have been proposed for how these complexes acquire and maintain their polarized localization, the machinery involved in moving core PCP proteins around cells remains unknown. We describe the AP-1 adaptor complex and Arf1 as major regulators of PCP protein trafficking in vivo . AP-1 and Arf1 disruption affects the accumulation of Fz/Fmi and Vang/Fmi complexes in the proximo–distal axis, producing severe PCP phenotypes. Using novel tools, we demonstrate a direct and specific Arf1 involvement in Fz trafficking in vivo . Moreover, we uncover a conserved Arf1 PCP function in vertebrates. Our data support a model whereby the trafficking machinery plays an important part during PCP establishment, promoting formation of polarized PCP-core complexes in vivo. Tissue organization requires highly ordered patterning and polarization of cells. Epithelial cells are frequently polarized within the following two axes: apical–basolateral (A/B) polarity and polarity within the plane of the epithelium, planar cell polarity (PCP). Acquisition and maintenance of polarity depends on the ability of a cell to traffic and maintain plasma membrane (PM) proteins in specific membrane domains. The PCP axis is established in part by highly conserved PCP-core complexes. Frizzled/Dishevelled/Diego (Fz/Dsh/Dgo) and Van Gogh/Prickle (Vang, a.k.a. Strabismus, Stbm/Pk) complexes localize to opposite PM domains within the same epithelial cell [1] , [2] , [3] , [4] , [5] , [6] . This mutually exclusive localization is reinforced by antagonistic interactions intracellularly and stabilizing intercellular interactions with adjacent cells [1] , [2] , [3] , [4] , [5] , [6] . The atypical cadherin Fmi (a.k.a. Starry night/Stan) completes the core group, it functions in both complexes, stabilizing them across membranes, and is required for Vang and Fz junctional/subapical membrane trafficking and/or stabilization [7] , [8] , [9] . In developing Drosophila wings, Fz/Dsh/Dgo/Fmi complexes are localized distally, whereas Vang/Pk/Fmi are localized proximally, relative to the body axis [3] . In adult wings, PCP manifests in the formation of a single distally pointing actin-based hair (trichome) per cell [10] . The core PCP factors acquire a robust planar-polarized localization from 6 h after pupa formation (APF) onwards [11] , [12] , [13] . Following cellular flow and rearrangements, the final proximo–distal (P–D)polarization emerges ∼ 28 h APF and ∼ 30 h APF, trichomes will start to form in a PCP-defined position and orientation [3] . Loss- and gain-of-function mutants of PCP components result in classical PCP phenotypes with defects in trichome number and/or orientation. These phenotypes have been used for screening of novel regulators of PCP complexes, as well as downstream effectors that link PCP-core signalling and actin dynamics, including mwh [14] , [15] , fuzzy [16] , inturned [17] , rho [18] , rock [19] , rac1 and cdc42 (refs 20 , 21 ). Although the core PCP PM proteins Fz, Vang and Fmi must be properly localized in epithelial cells, the trafficking molecules that are involved in their transport in vivo remain unknown. A recent study of the transport of Fz-PCP-core components suggested that the clathrin adaptor AP-1 and Arfaptin, a GTP-binding protein, might be required for the trafficking of Vangl2, a mouse Vang orthologue. The authors showed the requirement for these two trafficking proteins in the transport of Vangl2 from the trans-Golgi network (TGN) to the PM, but they used a non-polarized cell culture system and were therefore unable to analyse any PCP-related phenotypes [22] . Here, we identify Drosophila ADP ribosylation factor 1 (Arf1/Arf79F), a highly conserved trafficking-related GTPase, and its interactor, the AP-1 adaptor complex, as essential regulators of PCP-core component localization, producing PCP-specific defects in vivo . We demonstrate that perturbation of AP-1 and Arf1 function using RNA interference (RNAi), or blocking the GTP/GDP cycling of Arf1, caused characteristic PCP defects in multiple tissues. Importantly, this process appears to be conserved in vertebrates. Our data suggest that Arf1 is required for Fz trafficking during biosynthetic delivery, in vivo and in vitro , thus promoting Fz levels at the membrane and the formation of stabilized Fmi/Fz and Fmi/Vang complexes. Taken together, our data demonstrate that AP-1/Arf1 participate together to provide the correct levels and localization of Fz, Vang and Fmi in vivo . Loss-of-function of AP-1 causes PCP defects The AP-1 complex is a clathrin adaptor, working in the TGN and endosomes by recognizing and sorting cargo proteins into specific vesicles [23] . This hetero-tetrameric complex is composed of AP-1γ, AP-1β (shared with the endocytic clathrin adaptor AP-2 complex), AP-1 μ1 (also known as AP47) and AP-1σ subunits ( Supplementary Fig. 1d ). Using the engrailed -Gal4 ( en -Gal4, en >) driver and UAS-dsRNA sequences, we knocked down (KD) each of the subunits of the AP-1 complex in the posterior compartment of developing Drosophila wings, allowing direct comparison with the wild-type (WT) anterior compartment. KD of the large subunits of the complex, AP-1γ and AP-1β, resulted in lethality early in development at all temperatures tested. In contrast, KD of the smaller subunits of the complex, AP-1μ1 and AP-1σ, resulted in loss of tissue in the adult ( Fig. 1b,c compared with the control wing compartment, Fig. 1a ). Similar loss of tissue or very small wings were observed with other drivers such as nubbin- Gal4, which drives expression of dsRNA within the entire wing domain ( Supplementary Fig. 1a ). KD of the AP-1 subunits in the eye caused significant loss of tissue, making it difficult to reliably assess phenotypes from different genotypes, although clear PCP defects could be observed ( Supplementary Fig. 1b,c ). 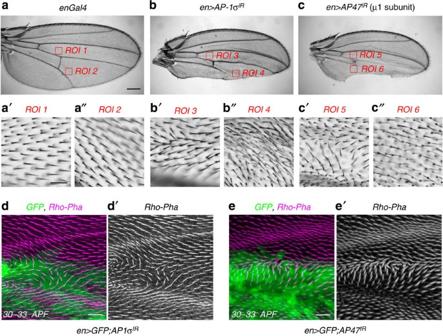Figure 1: AP-1μ1 and AP-1σ KD generate PCP phenotypes. (a) WT phenotype in adult wings expressingen-Gal4driver alone at low magnification ( × 5 image of whole wing). (b,c) KD of the AP-1σ and AP-1μ1 usingen-Gal4driver at × 5 magnification showed loss of tissue in the posterior domain, including margin defects. (b′,c′) Higher magnification ( × 20) of same wings fromb,crevealed PCP-related phenotypes, for example, mch and hair orientation defects, compared with the matching region of interest in a WT wing (a′). (b′′,c′′) More distal regions, closer to the margin of wings shown, displaying wing hair phenotypes in AP-1σIRand AP-1μ1IRgenotypes, including absence of hair or very thin hairs. (d–e′)en>AP47-IR oren>AP-1σ-IR (en-domain marked with GFP): note misorientation of actin-based wing hair (stained with rhodamine–phalloidin; magenta and monochrome ind′,e′). Scale bars, 250 μm (a–c); 25 μm (a′–c′′) and 10 μm (d,e′). Figure 1: AP-1μ1 and AP-1σ KD generate PCP phenotypes. ( a ) WT phenotype in adult wings expressing en-Gal4 driver alone at low magnification ( × 5 image of whole wing). ( b , c ) KD of the AP-1σ and AP-1μ1 using en-Gal4 driver at × 5 magnification showed loss of tissue in the posterior domain, including margin defects. ( b ′, c′ ) Higher magnification ( × 20) of same wings from b , c revealed PCP-related phenotypes, for example, mch and hair orientation defects, compared with the matching region of interest in a WT wing ( a ′). ( b ′′, c ′′) More distal regions, closer to the margin of wings shown, displaying wing hair phenotypes in AP-1σ IR and AP-1μ1 IR genotypes, including absence of hair or very thin hairs. ( d – e ′) en >AP47-IR or en >AP-1σ-IR ( en- domain marked with GFP): note misorientation of actin-based wing hair (stained with rhodamine–phalloidin; magenta and monochrome in d ′, e ′). Scale bars, 250 μm ( a – c ); 25 μm ( a ′– c ′′) and 10 μm ( d , e ′). Full size image Examined at higher magnification however, en -driven AP-1 σ KD or AP47 KD wings showed classical PCP-related phenotypes such as multiple cellular hairs (mch) and hair orientation defects ( Fig. 1b′ ). In addition other phenotypes were also apparent, including very thin hairs, crumpled tissue and margin defects ( Fig. 1b,b′′ and Supplementary Fig. 1a′ with nubbin-Gal4 ). PCP phenotypes were easier to score and analyse in pupal wings as these remained as flat epithelia. At 30–32 APF, KD of either of the small AP-1 subunits generated clear cellular hair misorientations and mch phenotypes (revealed by rhodamine–phalloidin staining; Fig. 1d,e′ ). In agreement with lethality and loss of tissue observed with the different dsRNAs against the AP-1 complex, clones of AP-1μ1 null mutant ( AP47 SHE11 ) cells in pupal wings were very small and only recoverable when induced at late stages of wing development (late third instar). These small AP-1μ1 null clones showed largely normal hair orientation and number ( Supplementary Fig. 1e–e′′ ), which likely reflects the persistence of AP-1μ1 protein under these conditions. In summary, our data on AP-1 loss-of-function using two dsRNAs against two distinct subunits of the complex showed robust PCP phenotypes in pupal wings. However, the widespread requirement for AP-1 and the loss-of-function phenotype being tissue and cell loss, most notably in adult wings and eyes, hindered a detailed analysis of the role of AP-1 complexes in establishing and maintaining PCP. Arf1 activity regulates PCP in various tissues Owing to the difficulties working with AP-1, we decided to look at known interactors of the AP-1 complex that promote its function and therefore might have a less severe yet related phenotype. One such interactor is ADP ribosylation factor 1 (Arf1 or Arf79F in Drosophila ), which is required for the conformational changes in the AP-1 complex that are needed for recognition of cargo proteins by the AP-1 complex itself ( Supplementary Fig. 1d ) [24] , [25] . There are no mutant alleles described for Arf1 in Drosophila. However, as Arf1 is a GTPase, its well-defined enzymatic function allows the use and study of GTP-locked (Arf1 Q71L ) and GDP-locked isoforms (Arf1 T31N ); in the case of trafficking, Arf1 must be able to cycle between GDP- and GTP-bound forms, and so both the GTP- and GDP-locked forms serve as functional interference tools [26] . Using the en -driver, we analysed effects of Arf1 Q71L and Arf1 T31N (ref. 27 ). Whereas expression of Arf1 T31N caused lethality at all temperatures tested, Arf1 Q71L induced both mch and PCP misorientation defects similar, but more specific, to those observed with AP-1 KDs ( Fig. 2a,a′ ). Overexpression of Arf1-WT did not cause PCP defects ( Fig. 7b ), supporting the idea that blocking GTP/GDP cycling has a specific inhibitory effect on Arf1 function. 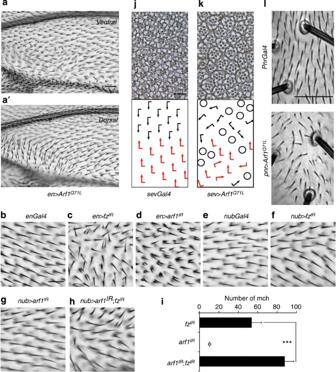Figure 2: Arf1 function is required for core PCP-mediated processes inDrosophila. (a,a′)en-Gal4 (en)>Arf1Q71Lgenerates mch and PCP hair orientation phenotypes on both sides of wing blade in posterior compartment. (b,c) WT phenotype in adult wings expressingen-Gal4driver alone and positive control ofen-driven Fz RNAi KD(en>fzIR) displaying hair orientation and mch phenotypes. (d) KD ofarf1gene caused strong mch phenotypes compared with WT control (b). (e–i) Genetic interactions betweenarf1andfzin adult wings. (f) Mild hair orientation and mch phenotypes are observed withnubbin-driven (nub-Gal4,nub>)fzIRcompared with WT control (e).nub>arf1IR(g) does not display mch phenotypes at 25 °C. (h) Double KD offzwitharf1enhances thefzIRphenotype. (i) Quantification of total mch number in the whole wing (n=10 wings). Columns represent the mean of mch and error bars represent the s.d.. ***P<0.001 (statistical analysis with Student’st-test). (j,k) Tangential sections of WT (j) andsev>Arf1Q71Leyes (k), which displays PCP phenotypes compared with WT control (j). Black and red arrows represent dorsal and ventral chiral ommatidia and circles represent ommatidia with R-cell loss; note also rotation defects in (k). (l–m)Pannier-driven expression of Arf1Q71Lcauses mch and hair orientation defects on the thorax (m) compared with WT control (l). Scale bars, 25 μm (a–h); 10 μm (j,k) and 50 μm (l,m). Figure 2: Arf1 function is required for core PCP-mediated processes in Drosophila . ( a , a ′) en-Gal4 (en)> Arf1 Q71L generates mch and PCP hair orientation phenotypes on both sides of wing blade in posterior compartment. ( b , c ) WT phenotype in adult wings expressing en-Gal4 driver alone and positive control of en -driven Fz RNAi KD (en>fz IR ) displaying hair orientation and mch phenotypes. ( d ) KD of arf1 gene caused strong mch phenotypes compared with WT control ( b ). ( e – i ) Genetic interactions between arf1 and fz in adult wings. ( f ) Mild hair orientation and mch phenotypes are observed with nubbin -driven ( nub- Gal4, nub> ) fz IR compared with WT control ( e ). nub>arf1 IR ( g ) does not display mch phenotypes at 25 °C. ( h ) Double KD of fz with arf1 enhances the fz IR phenotype. ( i ) Quantification of total mch number in the whole wing ( n =10 wings). Columns represent the mean of mch and error bars represent the s.d.. *** P <0.001 (statistical analysis with Student’s t -test). ( j , k ) Tangential sections of WT ( j ) and sev> Arf1 Q71L eyes ( k ), which displays PCP phenotypes compared with WT control ( j ). Black and red arrows represent dorsal and ventral chiral ommatidia and circles represent ommatidia with R-cell loss; note also rotation defects in ( k ). ( l – m ) Pannier -driven expression of Arf1 Q71L causes mch and hair orientation defects on the thorax ( m ) compared with WT control ( l ). Scale bars, 25 μm ( a – h ); 10 μm ( j , k ) and 50 μm ( l , m ). 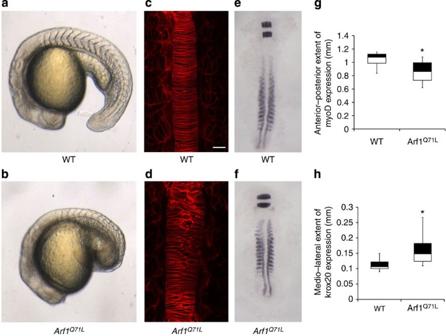Figure 3: Arf1 function is required for PCP-mediated processes in zebrafish. (a–h) Arf1 function during zebrafish embryogenesis. (a,b) Live lateral images of 18–19 somite stage embryos injected with 15 pg of WT Arf1 (a) and Arf1Q71L(b) mRNA. Arf1Q71Linjected embryos display lateral body curvatures and shortened AP and wider ML axes compared with WT controls. (c,d) Dorsal images of notochord cells labelled with membrane red fluorescent protein at 14–16 somite stage. (d) Arf1Q71Linjected embryos possessed 2–3-cell-thick columns consisting of both flattened and rounded cells compared with WT control (c). (e,f) Extent ofmyoDandkrox20expression in WT Arf1 (e) and Arf1Q71Lembryos (f) detected byin situhybridization. (g) Quantification of paraxial tissue AP length, measured by extent ofmyoDexpression, showing a significant reduction in paraxial tissue AP length of Arf1Q71Lembryos (n=27) compared with WT Arf1 (n=25), three independent experiments *P≤0.0001 (paired t-test). (h) Quantification of ML axes size, measured by extent ofkrox20expression in the fifthkrox20-positive rhombomere, indicating a significant increase in the size of ML axis of Arf1Q71Lembryos (n=27) compared with WT Arf1 (n=25), three independent experiments *P≤0.0001 (paired t-test). Error bars ing,hrepresent the min/max values of the data sets. Statistical analysis: Two-tailed pairedt-test. Scale bar, 20 μm. Full size image Figure 3: Arf1 function is required for PCP-mediated processes in zebrafish. ( a – h ) Arf1 function during zebrafish embryogenesis. ( a , b ) Live lateral images of 18–19 somite stage embryos injected with 15 pg of WT Arf1 ( a ) and Arf1 Q71L ( b ) mRNA. Arf1 Q71L injected embryos display lateral body curvatures and shortened AP and wider ML axes compared with WT controls. ( c , d ) Dorsal images of notochord cells labelled with membrane red fluorescent protein at 14–16 somite stage. ( d ) Arf1 Q71L injected embryos possessed 2–3-cell-thick columns consisting of both flattened and rounded cells compared with WT control ( c ). ( e , f ) Extent of myoD and krox20 expression in WT Arf1 ( e ) and Arf1 Q71L embryos ( f ) detected by in situ hybridization. ( g ) Quantification of paraxial tissue AP length, measured by extent of myoD expression, showing a significant reduction in paraxial tissue AP length of Arf1 Q71L embryos ( n =27) compared with WT Arf1 ( n =25), three independent experiments * P ≤0.0001 (paired t-test). ( h ) Quantification of ML axes size, measured by extent of krox20 expression in the fifth krox20 -positive rhombomere, indicating a significant increase in the size of ML axis of Arf1 Q71L embryos ( n =27) compared with WT Arf1 ( n =25), three independent experiments * P ≤0.0001 (paired t-test). Error bars in g , h represent the min/max values of the data sets. Statistical analysis: Two-tailed paired t -test. Scale bar, 20 μm. 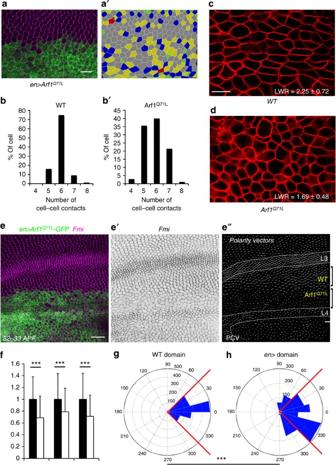Figure 4: Arf1Q71Lexpression generates PCP-specific defects. (a) Expression of Arf1Q71Lin the posterior compartment in the wing (marked by GFP) stained with anti-Fmi (same panel asFig. 5a). (a′) Using Fmi staining as the outline of cells (see Methods section) allows analysis of the number of cell–cell contacts, used as an indicative measurement of cell shape and cell packing in wing epithelia. (b) At 32–33 APF, cells in the WT region ofen>Arf1Q71Lwings display mainly a hexagonal shape, producing the classical hexagonal packing described for WT cells. (b′) In contrast, cells expressing Arf1Q71Ldisplay shapes of greater variation from a mean of six cell contacts, including a high percentage of pentagons and heptagons. (c,d) Zebrafish embryo dorsal ectoderm cells labelled with membrane red fluorescent protein from WT Arf1 (c) and Arf1Q71L(d) injected embryos at 90% epiboly, showing a reduced LWR for Arf1Q71Lembryos (1.68±0.48,n=270) compared with WT Arf1 embryos (2.25±0.72,n=306), three independent experimentsP≤0.0001. (e,e′) In pupal wings, polarized Fmi localization (magenta, monochrome ine′) is disrupted within the Arf1Q71Lexpression domain (marked by GFP, green). (e′′,f) Fmi staining is less polarized in Arf1Q71Lexpression area, and length of polarity vectors is reduced (quantified inffor three different wings). Columns for polarity vector lengths represent the mean length and s.d. error bars relative to WT. ***P<0.001 (Student’st-test). (g,h) Analyses of the polarity vector angles in veins and within the wing blade; note more variable polarity in Arf1Q71Lcells (n=1,488 cells from three different wings) compared with neighbouring WT control regions (n=1,285 cells from three different wings); ***P<0.001 (χ2-test). Scale bars, 10 μm (a,a′) 20 μm (e,e′′); 15 μm (c). Full size image Figure 4: Arf1 Q71L expression generates PCP-specific defects. ( a ) Expression of Arf1 Q71L in the posterior compartment in the wing (marked by GFP) stained with anti-Fmi (same panel as Fig. 5a ). ( a ′) Using Fmi staining as the outline of cells (see Methods section) allows analysis of the number of cell–cell contacts, used as an indicative measurement of cell shape and cell packing in wing epithelia. ( b ) At 32–33 APF, cells in the WT region of en> Arf1 Q71L wings display mainly a hexagonal shape, producing the classical hexagonal packing described for WT cells. ( b ′) In contrast, cells expressing Arf1 Q71L display shapes of greater variation from a mean of six cell contacts, including a high percentage of pentagons and heptagons. ( c , d ) Zebrafish embryo dorsal ectoderm cells labelled with membrane red fluorescent protein from WT Arf1 ( c ) and Arf1 Q71L ( d ) injected embryos at 90% epiboly, showing a reduced LWR for Arf1 Q71L embryos (1.68±0.48, n =270) compared with WT Arf1 embryos (2.25±0.72, n =306), three independent experiments P ≤0.0001. ( e , e ′) In pupal wings, polarized Fmi localization (magenta, monochrome in e ′) is disrupted within the Arf1 Q71L expression domain (marked by GFP, green). ( e ′′, f ) Fmi staining is less polarized in Arf1 Q71L expression area, and length of polarity vectors is reduced (quantified in f for three different wings). Columns for polarity vector lengths represent the mean length and s.d. error bars relative to WT. *** P <0.001 (Student’s t -test). ( g , h ) Analyses of the polarity vector angles in veins and within the wing blade; note more variable polarity in Arf1 Q71L cells ( n =1,488 cells from three different wings) compared with neighbouring WT control regions ( n =1,285 cells from three different wings); *** P <0.001 ( χ 2 -test). Scale bars, 10 μm ( a , a ′) 20 μm ( e , e ′′); 15 μm ( c ). 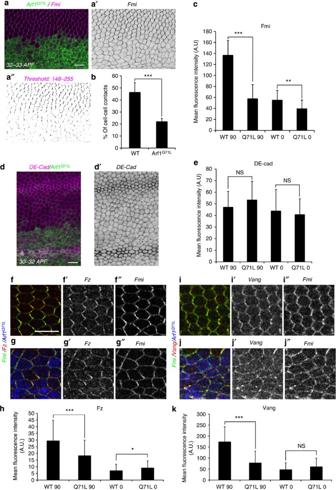Figure 5: Core PCP factor enrichment at cell membranes is reduced in Arf1Q71Lexpressing cells. (a–a′′) Wings expressing Arf1Q71Lshow decreased Fmi staining at junctions (magenta; monochrome ina′,a′′; (a′′) shows a rendering at a threshold cutoff of 148 grey value). (b) Quantification of percentage of cell–cell junctions with large puncta (strong Fmi staining), which is decreased in the Arf1Q71Lexpressing area. Columns represent percentage of cell–cell contacts with Fmi in large punctae. Error bars represent s.d.; ***P<0.001 (t-test). (c) Quantification of Fmi staining: note markedly reduced intensity in junctions close to 90° (relative to proximo–distal axis) in Arf1Q71Lexpression domain (Q71L 90) as compared with WT (WT 90), while Fmi intensity in junctions near 0° is only slightly affected (Q71L 0) compared with adjacent WT regions (WT 0). Bars represent mean fluorescence intensity and error bars represent s.d.. **P<0.01, ***P<0.001 (t-test). (d,e) DE-cadherin did not show differences between Arf1Q71Land WT regions (quantified ine; bars represent mean fluorescence intensity and error bars represent s.d.). (f–j′′) Fz (f–f′′ andg–g′; red, monochrome inf′,g′) and Vang (i–i′′ andj–j′′; red, monochrome inj′′) enrichment in proximal or distal junctional domains (close to 90°;n>75 cell–cell junctions from three areas) is reduced in Arf1Q71Lexpression domain, similar to Fmi (green, monochrome inf′′,g′′i′′,j′′). See alsoSupplementary Fig. 2for additional examples and cartoons indicating wing positions of presented areas. Quantification of Fz (h) and Vang (k) staining: note reduction in junctions close to 90° in Arf1Q71Lexpression domain (Q71L 90) as compared with WT (WT 90). Fz intensity in near 0° cell–cell contacts (n>40 cell–cell junctions from three areas) showed a minimal increase in Arf1Q71Lcells compared with WT regions (WT 0), while Vang was not changed (error bars represent s.d.’s). *P<0.05, ***P<0.001; NS, non-significant (all witht-test). Scale bars, 10 μm (for all panels). Full size image Figure 5: Core PCP factor enrichment at cell membranes is reduced in Arf1 Q71L expressing cells. ( a – a ′′) Wings expressing Arf1 Q71L show decreased Fmi staining at junctions (magenta; monochrome in a ′, a ′′; ( a ′′) shows a rendering at a threshold cutoff of 148 grey value). ( b ) Quantification of percentage of cell–cell junctions with large puncta (strong Fmi staining), which is decreased in the Arf1 Q71L expressing area. Columns represent percentage of cell–cell contacts with Fmi in large punctae. Error bars represent s.d. ; *** P <0.001 ( t -test). ( c ) Quantification of Fmi staining: note markedly reduced intensity in junctions close to 90° (relative to proximo–distal axis) in Arf1 Q71L expression domain (Q71L 90) as compared with WT (WT 90), while Fmi intensity in junctions near 0° is only slightly affected (Q71L 0) compared with adjacent WT regions (WT 0). Bars represent mean fluorescence intensity and error bars represent s.d.. ** P <0.01, *** P <0.001 ( t -test). ( d , e ) DE-cadherin did not show differences between Arf1 Q71L and WT regions (quantified in e ; bars represent mean fluorescence intensity and error bars represent s.d.). ( f – j ′′) Fz ( f – f ′′ and g – g ′; red, monochrome in f ′, g ′) and Vang ( i – i ′′ and j – j ′′; red, monochrome in j ′′) enrichment in proximal or distal junctional domains (close to 90°; n >75 cell–cell junctions from three areas) is reduced in Arf1 Q71L expression domain, similar to Fmi (green, monochrome in f ′′, g ′′ i ′′, j ′′). See also Supplementary Fig. 2 for additional examples and cartoons indicating wing positions of presented areas. Quantification of Fz ( h ) and Vang ( k ) staining: note reduction in junctions close to 90° in Arf1 Q71L expression domain (Q71L 90) as compared with WT (WT 90). Fz intensity in near 0° cell–cell contacts ( n >40 cell–cell junctions from three areas) showed a minimal increase in Arf1 Q71L cells compared with WT regions (WT 0), while Vang was not changed (error bars represent s.d.’s). * P <0.05, *** P <0.001; NS, non-significant (all with t -test). Scale bars, 10 μm (for all panels). 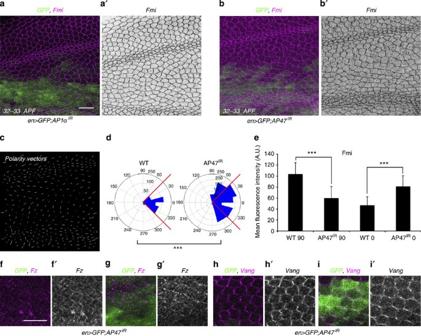Figure 6: The AP-1 complex KD disrupts the polarized pattern of core PCP complexes. (a) Polarized Fmi pattern (magenta and monochrome ina′) is disrupted in AP-1σ KD expression domain (marked with GFP ina). (b) Polarized Fmi pattern (magenta and monochrome inb′) is also disrupted inAP47-IRexpressing cells (marked with GFP inb). (c,d) Quantification of Fmi polarization using polarity vector angles; note variable polarization of Fmi in AP47 RNAi expressing cells (n=1,495 cells from three different wings) as compared with WT neighbouring cells (n=347 cells from three different wings); ***P<0.001 (χ2-test). (e) Quantification of Fmi staining in cell–cell contacts close to 90° and 0° (n>25 cell–cell junctions). Fmi staining is reduced in near 90° junctions inAP47-IRexpressing domain (KD 90) as compared with WT (WT 90). Fmi intensity in near 0° cell–cell contacts showed an increase in AP47 KD cells (KD 0) as compared with WT (WT 0). ***P<0.001; NS, non-significant (t-test). (f–i′) Fz (f,f′ andg,g′ magenta, monochrome inf′,g′) and Vang (h,h′ andi,i′ red, monochrome inh′,i′) enrichment proximal or distal junctional domains (close to 90°) is disrupted in AP47 KD expression domain (marked with GFP in green). Scale bars, 10 μm (for all panels). Full size image Figure 6: The AP-1 complex KD disrupts the polarized pattern of core PCP complexes. ( a ) Polarized Fmi pattern (magenta and monochrome in a ′) is disrupted in AP-1σ KD expression domain (marked with GFP in a ). ( b ) Polarized Fmi pattern (magenta and monochrome in b ′) is also disrupted in AP47-IR expressing cells (marked with GFP in b ). ( c , d ) Quantification of Fmi polarization using polarity vector angles; note variable polarization of Fmi in AP47 RNAi expressing cells ( n =1,495 cells from three different wings) as compared with WT neighbouring cells ( n =347 cells from three different wings); *** P <0.001 ( χ 2 -test). ( e ) Quantification of Fmi staining in cell–cell contacts close to 90° and 0° ( n >25 cell–cell junctions). Fmi staining is reduced in near 90° junctions in AP47-IR expressing domain (KD 90) as compared with WT (WT 90). Fmi intensity in near 0° cell–cell contacts showed an increase in AP47 KD cells (KD 0) as compared with WT (WT 0). *** P <0.001; NS, non-significant ( t -test). ( f – i ′) Fz ( f , f ′ and g , g ′ magenta, monochrome in f ′, g ′) and Vang ( h , h ′ and i , i ′ red, monochrome in h ′, i ′) enrichment proximal or distal junctional domains (close to 90°) is disrupted in AP47 KD expression domain (marked with GFP in green). Scale bars, 10 μm (for all panels). 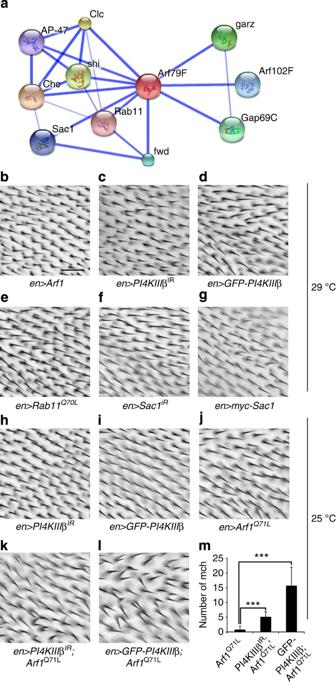Figure 7: Arf1 network cooperates in the establishment of PCP. (a) Arf1/Arf79F network, established using STRING software. (b) Arf1-WT overexpression in the wing does not generate PCP-related phenotypes. (c,d)PI4KIIIβinduces mch phenotypes. Both, KD of PI4KIIIβ (c) or overexpression of PI4KIIIβ (d) generate mch phenotypes, expressed withen-Gal4(en>) at 29 °C. (e) Mch formation inen>Rab11Q70Ladult wings. (f,g) KD of Sac1 (f) and overexpression of Sac1 (g) also both generate mch phenotypes, when expressed withen-Gal4(en>) at 29 °C. (h–l) PI4KIIIβ/Fwd enhances Arf1Q71L mch phenotypes.en-Gal4-mediated KD of PI4KIIIβ (h) or overexpression of PI4KIIIβ (i) do not generate mch phenotypes at 25 °C. Combination ofen>Arf1Q71L with PI4KIIIβ dsRNA (k) or overexpression of PI4KIIIβ (l) increased the number of mch in the posterior compartment as compared withen>Arf1Q71Lalone (j). (m) Mch defects were quantified in areas in the wing between L4 and L5, and the mean of the total number is presented. Error bars represent s.d. ***P<0.001 (Student’st-test),n=10. Scale bars, 25 μm (for all panels). Full size image Figure 7: Arf1 network cooperates in the establishment of PCP. ( a ) Arf1/Arf79F network, established using STRING software. ( b ) Arf1-WT overexpression in the wing does not generate PCP-related phenotypes. ( c , d ) PI4KIIIβ induces mch phenotypes. Both, KD of PI4KIIIβ ( c ) or overexpression of PI4KIIIβ ( d ) generate mch phenotypes, expressed with en-Gal4 ( en> ) at 29 °C. ( e ) Mch formation in en >Rab11 Q70L adult wings. ( f , g ) KD of Sac1 ( f ) and overexpression of Sac1 ( g ) also both generate mch phenotypes, when expressed with en-Gal4 ( en> ) at 29 °C. ( h – l ) PI4KIIIβ/Fwd enhances Arf1Q71L mch phenotypes. en- Gal4-mediated KD of PI4KIIIβ ( h ) or overexpression of PI4KIIIβ ( i ) do not generate mch phenotypes at 25 °C. Combination of en> Arf1Q71L with PI4KIIIβ dsRNA ( k ) or overexpression of PI4KIIIβ ( l ) increased the number of mch in the posterior compartment as compared with en> Arf1 Q71L alone ( j ). ( m ) Mch defects were quantified in areas in the wing between L4 and L5, and the mean of the total number is presented. Error bars represent s.d. *** P <0.001 (Student’s t -test), n =10. Scale bars, 25 μm (for all panels). Full size image To confirm this and to directly compare with AP-1 KD, we KD Arf1 in the posterior compartment of developing Drosophila wings, using the en -Gal4, en > driver and UAS-dsRNA sequences ( Fig. 2d ). As controls, RNAi mediated Fz KD ( fz IR ) affected both the number and orientation of cellular hairs, and en -Gal4 alone had no effect ( Fig. 2b,c ). Arf1 dsRNA ( Arf1 IR ) wings displayed strong mch and orientation phenotypes at 29 °C ( Fig. 2d ). Taking advantage of the observation that Arf1 IR wing phenotypes were weaker at lower temperatures, we used Arf1 IR to test for genetic interactions with the PCP-core component Fz. KD of Fz with nubbin- Gal4 ( nub>fz IR , expressed throughout the wing pouch) generated both hair orientation and mch defects, whereas nub>Arf1 IR had no effect under these conditions ( Fig. 2f, g ). Combining the Arf1 and Fz KDs strongly enhanced the fz IR phenotype ( Fig. 2h ): with the Arf1 IR and fz IR combination enhancing orientation defects and almost doubling the number of mch defects per wing as compared with fz IR alone ( Fig. 2f–i ). To investigate whether the Arf1 PCP phenotypes were more wide ranging, we examined other tissues in which AP-1 was difficult to study due to its associated cell lethality. The adult eye comprises a regular array of photoreceptor clusters, ommatidia, whose orientation and chirality are directly established by core PCP factors [28] , [29] . The sevenless -Gal4 ( sev> ) driver is expressed transiently in the two R-cells [R3/R4] that are critical for PCP establishment. sev >Arf1 Q71L expression caused PCP defects including misrotated ommatidia and chirality defects, as well as loss of photoreceptors ( Fig. 2j,k , quantified in Supplementary Fig. 2d ). This was confirmed with sev>Arf1 IR KD eyes that displayed a similar phenotype ( Supplementary Fig. 2b,d ). Strikingly, Arf1 T31N , which was lethal with other drivers, yielded adult flies with sev -promoter-driven expression, displaying severe PCP chirality and orientation defects ( Supplementary Fig. 2c,d ). Similarly, we observed classical PCP defects with Arf1 Q71L in the thorax, within the pannier ( pnr ) Gal4 expression domain, displaying cellular polarity defects and mch phenotypes ( Fig. 2l,m ). Taken together, these results indicate that Arf1 is a general regulatory factor of PCP establishment in Drosophila . In summary, loss of function of Arf1 using different interference tools caused classical PCP defects in the wing, eye and thorax. Phenotypes that, at least in the wing, were reminiscent of those observed in loss-of-function scenarios of AP-1μ1 and AP-1σ from the AP-1 complex. Importantly, we were also able to demonstrate a strong genetic interaction of Arf1 with the PCP-core component Fz. Evolutionary conserved function of Arf1 in PCP Arf1 is a highly conserved protein with over 90% amino-acid identity from yeast to humans, including plants. To investigate whether Arf1 PCP function(s) were conserved, we examined the requirement for Arf1 in zebrafish development. We evaluated the consequence of hArf1-WT or hArf1 Q71L expression on embryonic patterning and morphogenesis. In vitro synthesized capped mRNA encoding each hArf1 form were injected into WT embryos at the one-cell stage, at amounts ranging from 10 to 120 pg. At all concentrations examined, hArf1-WT produced no obvious developmental phenotypes ( Fig. 3a and not shown). In contrast, as little as 20 pg of hArf1 Q71L mRNA was toxic to the embryo. At 15 pg of hArf1 Q71L mRNA, 78% of injected embryos ( n =114) developed lateral body curvatures and had shortened anterior–posterior (AP) and widened medio–lateral (ML) axes, consistent with defects in PCP ( Fig. 3b ). To further determine the role for Arf1 in axial morphogenesis, we examined notochord formation in hArf1-WT and hArf1 Q71L -injected embryos ( Fig. 3c,d ). Beginning late in gastrulation, the axial mesoderm narrows to form a two-cell-wide column running along the AP axis of the developing embryo, which then undergoes further PCP-directed cell intercalations to form a single stack of notochord cells [30] . While the notochord of WT-hArf1 embryos appeared normal ( Fig. 3c ), notochords of hArf1 Q71L embryos remained as 2–3-cell-thick columns, exhibiting both flattened and rounded cell types ( Fig. 3d ). These defects are consistent with abnormal PCP-directed convergence and extension (CE) movements. To quantify axial morphogenesis defects in hArf1 Q71L embryos, we performed morphometric analyses of myoD and krox20 expression in hArf1-WT versus hArf1 Q71L embryos at the 14-somite stage ( Fig. 3e–h ). The AP length of paraxial mesoderm in hArf1 Q71L embryos was significantly reduced, as measured by the extent of myoD expression within the trunk of the embryo ( Fig. 3g ). In addition, the size of the ML axis of the hArf1 Q71L embryos significantly increased, as measured by the width of the fifth rhombomere stained with krox20 ( Fig. 3h ). In summary, hArf1 Q71L -injected embryos demonstrate significant disruptions in axial morphogenesis, phenotypes typically observed in core PCP signalling mutants [31] , [32] , and we thus conclude that Arf1 could play a conserved role in PCP establishment from Drosophila to vertebrates. Arf1/AP-1 function is required for proper cell shape Cell junction remodelling is an important feature of PCP establishment. Cells need to rotate, migrate and intercalate in order to acquire the right packing within a tissue. In Drosophila, these cellular packing phenotypes are in part resolved by core PCP proteins and this feature is an established PCP-associated wing defect [33] . When examining cellular packing in pupal wings of Arf1 and AP-1 interference mutants, we observed that Arf1 Q71L as well as AP-1μ1 KD caused packing defects of wing cells ( Fig. 4a,a′’ ; quantified in Fig. 4b,b′ and Supplementary Fig. 3a–c ). Both conditions resulted in fewer cells with hexagonal cell shape (six cell–cell contacts) as compared with the adjacent WT region of same wings ( Fig. 4a,b′ and Supplementary Fig. 3a–c ). Similar to Drosophila wing cell packing, core PCP factors affect cell shape changes during vertebrate gastrulation and CE processes. For example, dorsal ectoderm cells undergoing PCP-directed CE movements elongate along the ML axis as they migrate towards the embryo midline, and PCP-core factor function is required for this elongation [31] , [32] . Consistent with a conserved function of Arf1 in vertebrate PCP, the length-to-width ratio (LWR) of dorsal ectoderm cells in hArf1 Q71L -injected embryos was significantly reduced compared with that of WT Arf1 cells ( Fig. 4c,d ). These data confirm a conserved Arf1 function early during PCP establishment, and establish that the Arf1 and AP-1 PCP defects are very similar to those observed with core PCP factor mutants in terms of cell shape and packing. Arf1 is required for formation of polarized PCP complexes The planar-polarized subcellular localization differences of the core PCP factors are early evidence of PCP within a tissue, and are best studied in pupal wings. In this tissue, the different complexes can be visualized as a characteristic ‘zig-zag’ pattern with enrichment of Fmi, Fz and Vang in the P–D axis. Thus, we first confirmed the presence of the PCP defects observed in the adult at this earlier stage, analysing the pupal wing epithelia of en>Arf1 Q71L flies with anti-Fmi staining. Whereas in WT wings at 30–32 h APF, when the core PCP factors form the PCP-specific zig-zag pattern in the P–D axis, in the Arf1 Q71L wings the polarized pattern of Fmi was lost ( Fig. 4e,e′ ; compared to WT/anterior wing domain). Polarity can be quantified by measuring polarity vector length (nematic order) and angle based on polarized Fmi staining (see Methods section; ref. 11 ). Nematic order decreased over 25% from WT to Arf1 Q71L ( Fig. 4e′′ ). Moreover, not only was polarity strength diminished but also the vector angles became irregular in Arf1 Q71L relative to WT ( Fig. 4e′′ , quantified in Fig. 4g,h ). In agreement with the adult phenotypes, en > Arf IR cause a modest but significant defect in Fmi staining and angle distribution in pupal wings ( Supplementary Fig. 3d–g ). Similar Fmi staining defects were observed in Arf1 Q71L expressing clones and, importantly, also surrounding WT cells ( Supplementary Fig. 3h–h′′′ ), reflecting the expected non-autonomous effects similar to fz - clones (or fmi -, fz or Vang-, fz- double mutant clones [34] , [35] , [36] ; note that Fmi protein reduction in Arf1 Q71L expressing cells is detected from early third instar stage onwards, for example, in the posterior compartment; Supplementary Fig. 3i,j ). Polarized localization of Fz/Fmi and Vang/Fmi complexes at P–D cell–cell junctions is due to the formation of stable puncta, which are resistant to endocytosis and necessary for proper PCP patterning [13] . Fmi localization was (i) largely unpolarized in the Arf1 Q71L expressing domain and (ii) the levels of Fmi were reduced ( Figs 4e,e′ and 5a,a′ ). Specifically, the larger junctional Fmi puncta were significantly reduced as compared with the adjacent WT domain ( Fig. 5a′′ ). Since Arf1 controls trafficking of PM proteins, we asked whether protein levels at the PM were reduced in general, or whether this was a specific effect on Fmi (and/or other core PCP factors). We therefore quantified cell–cell contact protein levels of Fmi, DE-cadherin and FasIII by immunofluorescence. Fmi levels at cell–cell junctions close to a 90° angle (perpendicular to the P–D axis) were markedly reduced ( Fig. 5c ; to less than half in Arf1 Q71L expressing cells as compared with WT control cells), as suggested by the polarity vector length quantifications ( Fig. 4e′′ ). In contrast, cell–cell junction staining of Fmi at cell contacts close to 0° angle were only slightly affected in Arf1 Q71L expressing cells ( Fig. 5c ), suggesting a specific effect on P–D-localized complexes. Accordingly, DE-cadherin and FasIII localization analyses showed no changes at junctional levels or at the basolateral membrane, respectively ( Fig. 5d,e and Supplementary Fig. 4a,b , and xz views in Supplementary Fig. 4m–n′′ ). Taken together, these data indicated that a disruption of Arf1 function specifically abolished the enrichment of Fmi in polarized complexes along P–D junctional domains. Next, we examined Fz and Vang localization. Similar to Fmi, both were reduced at P–D junctional areas (90° angle) in Arf1 Q71L expressing cells but were not affected in AP junctional domains. The puncta staining was markedly reduced for Fz in cell–cell junctions close to the 90° angle and minimally increased in those close to 0° angle contacts ( Fig. 5f–h and Supplementary Fig. 4c–j ). Vang also displayed a very similar changed pattern, such as Fz, in cells expressing Arf1 Q71L , as compared with WT cells ( Fig. 5i–k and Supplementary Fig. 4h–l ). In summary, interference with Arf1 function specifically affects the planar-polarized enrichment of the core PCP factors Fmi, Fz and Vang, with no effect on the other PM proteins tested. AP-1 affects polarized localization of core PCP complexes As mentioned above, the function of AP-1 is to directly recognize and sort cargo proteins into specific vesicles [23] . In Drosophila , Le Borgne and colleagues [37] have shown that the Notch regulator Sanpodo is regulated by AP-1 with no effect on general A/B transport of DE-cadherin and FasIII in the notum. In the wing, en -driven AP47 dsRNA or AP-1σ dsRNA showed non-polarized Fmi staining quantified by polarity vector angle distribution ( Fig. 6a–d ), similar to what we have observed for Arf1 Q71L expressing cells (see Fig. 4e–h for comparison). However, we did not observe the general reduction in Fmi membrane staining detected in en>Arf1 Q71L wings when analysed for fluorescence intensity in junctions close to 90 or 0 degrees ( Fig. 6e ; note non-polarized). A similar staining pattern was observed for Vang and Fz in AP47-IR cells ( Fig. 6f–i′ ). In general, AP-1 loss of function produced phenotypes very similar to Arf1 Q71L expressing cells, with Fmi, Fz and Vang not properly polarized in the P–D axis (for example, Fig. 6e , with the difference between WT 90 and WT 0 that reflects polarity being lost in the mutant cells, and AP47 IR -90 and AP47 IR -0 displaying very similar values). The difference between en -driven AP47 dsRNA or AP-1σ dsRNA and Arf1 Q71L is that overall Fmi levels are not affected in AP-1 KDs, whereas there is less Fmi in Arf1 Q71L cells. This might reflect an additional function of Arf1 in other trafficking steps, for example, together with COPI in the retrograde transport out of the Golgi (see Discussion section). The Arf1 protein network displays PCP-related phenotypes To better understand the molecular mechanism by which AP-1 and Arf1 function in PCP establishment and identify other proteins involved, we analysed members of the Arf1 protein interaction network ( Fig. 7a ). One candidate that stood out was phosphatidylinositol 4-kinase III beta (PI4KIIIβ; Four wheel drive/Fwd in Drosophila ). We had previously isolated PI4KIIIβ/Fwd in an independent genetic screen for new PCP regulators, in which we showed that fwd mutants displayed PCP phenotypes in Drosophila eyes and wings [38] . Arf1 also regulates PI4KIIIβ localization in the Golgi [39] , and together PI4KIIIβ and Arf1 recruit adaptor proteins such as the AP-1 complex, which is required for budding and cleavage of Golgi-derived vesicles [40] . Manipulation of PI4KIIIβ/fwd levels in the developing wing, using en -driven PI4KIIIβ dsRNA or GFP-PI4KIIIβ expression, leads to a mch phenotype ( Fig. 7c,d ). This phenotype was confirmed in PI4KIIIβ Z0453 mutant clones in pupal wings, which showed mch defects (detected by F-actin staining in developing hairs with rhodamine–phalloidin; Supplementary Fig. 6a,a′ ). These results prompted us to test genetic interactions between Arf1 and PI4KIIIβ . At 25 °C, en>PI4KIIIβ-IR and en>GFP-PI4KIIIβ do not display mch phenotypes ( Fig. 7h,i ). In the same wing region, en -driven Arf1 Q71L caused hair orientation defects but almost no mch ( Fig. 7j ). Importantly, when Fmi staining was analysed at 25 °C, the combination of Arf1 Q71L and PI4KIIIβ-IR enhanced the Arf1 Q71L phenotype in terms of polarity vector angle distribution ( Supplementary Fig. 5j–o and Supplementary Table 1 ). In contrast, we did not observe any significant genetic interaction between Arf1 Q71L and GFP-PI4KIIIβ ( Supplementary Fig. 5p–u and Supplementary Table 1 ). Furthermore, co-expression of PI4KIIIβ-IR or GFP-PI4KIIIβ with Arf1 Q71L resulted in a significant increase of mch ( Fig. 7k–m : from an average of 0.7 mch in Arf1 Q71L alone to 5 and 15.6 mch, respectively), suggesting that these factors function together during the manifestation of PCP. We next investigated two other components of the Arf1 network: Sac1 and Rab11. Sac1 is the phosphatase that catalyses the inverse reaction to PI4KIIIβ. PI4KIIIβ has been shown to bind and recruit the GTP-bound form of Rab11, overexpression of which leads to the formation of mch in the wing [41] . Expression of Rab11 Q70L or Sac1 at 29 °C lead to a mch phenotype that was similar to that observed when manipulating PI4KIIIβ levels ( Fig. 7e–g ). However, when Fmi staining was analysed, Rab11 Q70L did not show Fmi staining defects in angle distribution or polarity vector length at 29 °C ( Supplementary Fig. 5g–i ), nor did we observe any significant genetic interaction between Arf1 Q71L and Rab11 Q70L ( Supplementary Fig. 5p–u ). Taken together, our data on Arf1 and AP-1 strongly suggest that these two factors are directly involved in the transport of PCP-core proteins during PCP establishment. Moreover, other components of the Arf1 network, Rab11, Sac1 and PI4KIIIβ, also appear to play a role in PCP. Whereas Rab11 and Sac1 are more likely to act as effectors downstream of the core PCP receptors, PI4KIIIβ appears to function together with AP-1/Arf1 in PCP-core factor trafficking. Arf1/PI4KIIIβ/Rab11 partially co-localize with AP-1 Generally, the Arf1/AP-1 protein network ( Fig. 7a ) is required both at the Golgi and endosomes, promoting trafficking towards the PM [23] , [42] , [43] . To better define the compartment where Arf1 and AP-1 were interacting, we analysed the cellular localization of Arf1, AP-1 and PI4KIIIβ during PCP-associated processes. Analysis during PCP establishment up to the pre-hair/hair formation stages in pupal wings confirmed that at all times Arf1 is localized in intracellular organelles, as are AP-1 components and PI4KIIIβ ( Fig. 8b,d,f and Supplementary Fig. 6b–d ). At later stages (32–33 APF), enrichment of Arf1, AP-1 and PI4KIIIβ was also observed in emerging hairs, while their localization did not change in other areas of the cell ( Fig. 8a,c,e showing apical focal planes; and Fig. 8b,d,f showing subapical planes). When tested for co-localization, partial overlap was observed between Arf1 and AP-1 ( Fig. 8g ) or PI4KIIIβ and AP-1 ( Fig. 8h ). Consistent with the notion that Arf1 also affects other processes, only a subset of the Arf1- or PI4KIIIβ-positive punctae were decorated with AP-1. 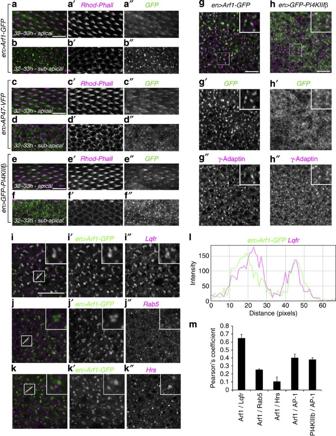Figure 8: Arf1, AP-1, PI4KIIIβ and Rab11 co-localizein vivoand in cultured cells. (a–f′′) Localization of Arf1 (GFP tagged; green and monochrome) (a′′,b′′) AP47 (VFP tagged, green and monochrome) (c′′,d′′) or PI4KIIIβ (GFP tagged, green and monochrome) (e′′,f′′ and actin (co-stained with rhodamine–phalloidin (red and monochrome) (a′–f′) in pupal wings during hair formation (32–33 h APF). Arf1, AP47 and PI4KIIIβ are enriched in the hair (a′′,c′′,e′′) and localize in a puncta pattern in subapical planes (b′′,d′′,f′′). (g) Arf1 (g′) and γ-adaptin (g′′) partial co-localization in pupal wings, upper right corner shows high magnification of puncta co-localizion. (h) PI4KIIIβ (h′) and γ-adaptin (h′′) also partially co-localize in pupal wings, upper right corner shows high magnification of co-localizing puncta. (i–k) Arf1 shows high co-localization with LqfR (i) but very little co-localization with Rab5 (j) or Hrs (k). For co-localization analyses, line profile (l) and Pearson’s coefficients were calculated (m), error bars represent s.d. ***P<0.001 (t-test). Scale bars, 10 μm. Figure 8: Arf1, AP-1, PI4KIIIβ and Rab11 co-localize in vivo and in cultured cells. ( a – f ′′) Localization of Arf1 (GFP tagged; green and monochrome) ( a ′′, b ′′) AP47 (VFP tagged, green and monochrome) ( c ′′, d ′′) or PI4KIIIβ (GFP tagged, green and monochrome) ( e ′′, f ′′ and actin (co-stained with rhodamine–phalloidin (red and monochrome) ( a ′– f ′) in pupal wings during hair formation (32–33 h APF). Arf1, AP47 and PI4KIIIβ are enriched in the hair ( a ′′, c ′′, e ′′) and localize in a puncta pattern in subapical planes ( b ′′, d ′′, f ′′). ( g ) Arf1 ( g ′) and γ-adaptin ( g ′′) partial co-localization in pupal wings, upper right corner shows high magnification of puncta co-localizion. ( h ) PI4KIIIβ ( h ′) and γ-adaptin ( h ′′) also partially co-localize in pupal wings, upper right corner shows high magnification of co-localizing puncta. ( i – k ) Arf1 shows high co-localization with LqfR ( i ) but very little co-localization with Rab5 ( j ) or Hrs ( k ). For co-localization analyses, line profile ( l ) and Pearson’s coefficients were calculated ( m ), error bars represent s.d. *** P <0.001 ( t -test). Scale bars, 10 μm. Full size image Co-localization studies with endosomes and TGN markers reveal that the majority of Arf1 was present in intracellular structures co-stained with LqfR (a known TGN marker [44] ), as shown by line profile analyses and by the Pearson’s correlation coefficient ( Fig. 8i–i′′ ). Very little co-localization was observed between Arf1 and Rab5 (early endosomes) or Hrs (multivesicular bodies) as shown by the Pearson’s correlation coefficients and line profiles ( Fig. 8j–m and Supplementary Fig. 6e,f ). Co-expression of Arf1 and PI4KIIIβ and staining for the AP-1γ (γ−adaptin) subunit of the AP-1 complex in S2 cells revealed the same pattern observed in vivo , showing partial co-localization between Arf1 and AP-1 or PI4KIIIβ and AP-1 ( Supplementary Fig. 6g–g′′′ ). On the other hand, almost perfect overlap was observed for Arf1 and PI4KIIIβ ( Supplementary Fig. 6g–g′′ ). This was also the case for Arf1 and Rab11 or PI4KIIIβ and Rab11 ( Supplementary Fig. 6h–h′′′ ). Taken together, these data define where in the trafficking process the core PCP proteins are recognized by AP-1 and Arf1: a compartment with TGN molecular features containing Arf1/PI4KIIIβ/Rab11 and decorated with AP-1. Arf1 controls Fz trafficking in vitro and in vivo As interference with Arf1 function caused defects in the junctional accumulation of PCP proteins into polarized complexes, we investigated whether Arf1 is required for the delivery of PCP proteins to the PM. To do so, we adapted a method originally established by Rivera et al. [45] , [46] , [47] to study biosynthetic delivery of proteins using a drug-inducible system to synchronize trafficking events, the iDimerize Reverse Dimerization System (see Methods section). This system is based on the dimerization property of the DmrD domains [45] , [46] , [47] . In the absence of the drug, D/D solubilizer, the chimeric proteins containing the DmrD dimerization domain remain in the endoplasmic reticulum (ER) due to their aggregation. Upon drug addition, the protein disaggregates and can be trafficked through its normal biosynthetic pathway ( Fig. 9a,a′ ). We first established that this method was suitable for PM protein delivery in Drosophila S2 cells and in vivo, and then used it to address Arf1 function in the trafficking of Fz, the structurally best characterized [48] , [49] of the three core PCP PM proteins. We generated a Drosophila Fz construct with a myc-epitope tag in the extracellular domain [48] , in frame with four DmrD domain repeats ( Fig. 9a,a′ ). In Drosophila S2 cells, in the absence of the disaggregating drug, the chimeric Fz protein (DmrD4-Fz-GFP) remains stuck in the ER with minimal levels at the PM ( Fig. 9a,b ). Upon addition of the D/D solubilizer (release from ER), Fz is detected at high levels at the PM within 120–180 min ( Fig. 9a,c–c′′ ). PM arrival was confirmed by immunofluorescence without permeabilization (against the extracellular myc-epitope in Fz; Fig. 9c′′ ). In addition, treatment of S2 cells with Brefeldin A (BFA; an inhibitor of Arf1-GEFs typically associated with biosynthetic transport that does not affect the PM Arf1-GEFs) or KD of Arf1 by dsRNA markedly reduced arrival of the chimeric Fz protein at the PM ( Fig. 9d–d′′ ), with BFA almost completely blocking Fz traffic. 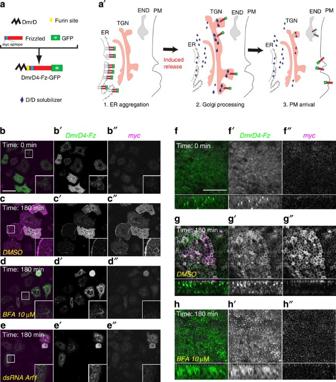Figure 9: Arf1 controlsde novoFz trafficking to the membrane. (a,a′) Schematic representation of the construct pAc-DmrD4-Fz-GFP (a) and the cellular pathway that the protein follows after release with D/D Solubilizer (a′). ER, TGN, endosomes (END) and PM. The molecular cloning and strategy are described in Methods section. (b–e′′) Trafficking of pAc-DmrD4-Fz-GFP in S2 cells. (b–b′′) Transfection of pAc-DmrD4-Fz-GFP in S2 cells with accumulation in the ER (b,b′) and no detectable Fz chimera at the membrane in non-permeabilized cells (b′′), lower right corner shows single cell in high magnification. (c–c′′) Following D/D solubilizer drug treatment, DmrD4-Fz-GFP is trafficked to the membrane, as shown by anti-myc immunofluorescence without permeabilization (high magnification in lower right corner;c′′). (d–e′′) BFA treatment (d–d′′ or dsRNA against Arf1 (e–e′′) markedly reduces Fz trafficking to the PM after D/D solubilizer drug treatment (single-cell high magnification in lower right corner). (f–h′′) Trafficking of pAc-DmrD4-Fz-GFPin vivo. Bottom panels show X-Z sections of the respective panels above. (f–f′′) Expression of DmrD4-myc-Fz-GFPin vivoin third instar wing discs showed aggregation of Fz in the ER before D/D solubilizer drug treatment, with hardly any detectable extracellular myc staining (f′′ without permeabilization). (g–g′′) Within 180 min of D/D solubilizer treatment, Fz is trafficked to junctional membrane regions and detected with anti-myc antibody without permeabilization (g′′; note also subapical junctional localization of Fz in X-Z section, bottom panel ofg′′). (h–h′′) Arf1 inhibition via BFA treatment impairs Fz trafficking to the membrane, as little membrane staining can be detected using anti-myc antibody (h′′, see also bottom panel for X-Z section). Scale bars, 25 μm. Figure 9: Arf1 controls de novo Fz trafficking to the membrane. ( a , a ′) Schematic representation of the construct pAc-DmrD4-Fz-GFP ( a ) and the cellular pathway that the protein follows after release with D/D Solubilizer ( a ′). ER, TGN, endosomes (END) and PM. The molecular cloning and strategy are described in Methods section. ( b – e ′′) Trafficking of pAc-DmrD4-Fz-GFP in S2 cells. ( b – b ′′) Transfection of pAc-DmrD4-Fz-GFP in S2 cells with accumulation in the ER ( b , b ′) and no detectable Fz chimera at the membrane in non-permeabilized cells ( b ′′), lower right corner shows single cell in high magnification. ( c – c ′′) Following D/D solubilizer drug treatment, DmrD4-Fz-GFP is trafficked to the membrane, as shown by anti-myc immunofluorescence without permeabilization (high magnification in lower right corner; c ′′). ( d – e ′′) BFA treatment ( d – d ′′ or dsRNA against Arf1 ( e – e ′′) markedly reduces Fz trafficking to the PM after D/D solubilizer drug treatment (single-cell high magnification in lower right corner). ( f – h ′′) Trafficking of pAc-DmrD4-Fz-GFP in vivo . Bottom panels show X-Z sections of the respective panels above. ( f – f ′′) Expression of DmrD4-myc-Fz-GFP in vivo in third instar wing discs showed aggregation of Fz in the ER before D/D solubilizer drug treatment, with hardly any detectable extracellular myc staining ( f ′′ without permeabilization). ( g – g ′′) Within 180 min of D/D solubilizer treatment, Fz is trafficked to junctional membrane regions and detected with anti-myc antibody without permeabilization ( g ′′; note also subapical junctional localization of Fz in X-Z section, bottom panel of g ′′). ( h – h ′′) Arf1 inhibition via BFA treatment impairs Fz trafficking to the membrane, as little membrane staining can be detected using anti-myc antibody ( h ′′, see also bottom panel for X-Z section). Scale bars, 25 μm. Full size image Next, we generated flies expressing DmrD4-Fz-GFP chimeras under nub -Gal4 control and examined the effect of Arf1 on Fz trafficking in vivo in third instar wing discs. Before drug addition, DmrD4-Fz-GFP protein was stuck in the ER and almost undetectable at the PM ( Fig. 9f–f′′ ). In contrast, after 180 min of D/D solubilizer treatment-mediated release, DmrD4-Fz-GFP arrived at the membrane, acquiring the normal Fz-localization at apical junctional regions ( Fig. 9g–g′′ ). Co-treatment with the Arf1 inhibitor BFA largely abolished the delivery of the Fz fusion protein to apical junctional regions ( Fig. 9h-h” ). Under these same conditions, DE-cadherin staining was not perturbed ( Supplementary Fig. 7 ). Taken together, these experiments demonstrate that Arf1 controls the trafficking of newly synthesized Fz to the PM to allow Fz enrichment in junctional regions, both in vitro and in vivo in developing Drosophila wings. Here we demonstrate that the AP-1 complex and Arf1 are critical for PCP-core protein membrane localization during PCP establishment in multiple Drosophila tissues, and that it likely serves as a conserved function in zebrafish. Detailed analysis in Drosophila wings and zebrafish cells during gastrulation revealed that Arf1 function is required for polarized accumulation of core PCP components during PCP axis establishment. Defects in correct planar-polarized localization resulted in classical PCP defects in both animal models, and thus our study reveals a conserved function of the Arf1 protein network. Arf1 and AP-1 act as the trafficking machinery for the core PCP components in epithelial cells during PCP establishment. A few studies suggested connections between PCP and trafficking before. First Rabenosyn, an endocytic-related protein, was found polarized in a PCP-type fashion following Fmi localization. Rabenosyn mutant cells display defects in cellular packing and accumulation of PCP-core components at the PM [50] . Second, the GTPase Rab23, which, similar to Rabenosyn, causes packing defects and mch, interacts with the cytosolic PCP-core protein Pk (ref. 51 ). And third, Gish/Rab11/nuf were recently shown to affect hair formation by either increasing the numbers of trichomes per cell (mch) or shortening the hairs (stunted hair phenotype) [41] . However, none of these proteins affected PCP-core component localization, including Fmi or Fz, or hair orientation in the adult, similar to the Arf1/AP-1 network does. Arf1 is known to act during trafficking from the Golgi in Drosophila and vertebrate cells. In the TGN, Arf1 aids in sorting of cargo proteins into carrier vesicles, regulating the binding of clathrin adaptor proteins such as GGAs (Golgi-localized, γ-adaptin ear-containing and ARF-binding proteins) or the clathrin adaptor complex AP-1 (refs 23 , 25 , 43 ). We demonstrate that perturbation of Arf1 and AP-1 function reduced polarized accumulation of Fmi, Fz and Vang with minimal effects on non-planar-polarized membrane proteins (for example, DE-cadherin and FasIII; also ref. 37 ). A distinct subpopulation of PCP-core component complexes with different turnover dynamics from unpolarized membrane junctional domains has recently been identified [13] . These complexes are polarized, stable and restricted to large puncta, and also insensitive to manipulations of the endocytic/recycling machinery [13] . Together with established Arf1/AP-1 functions at the Golgi, our data support the notion that stable PCP complexes originate mainly from newly synthesized PM proteins. A hypothesis that is further supported by using the DmrD4-Fz-GFP fusion and manipulations to synchronize its ER release. Inhibition of Arf1 with BFA treatment prevented the arrival of Fz to the membrane in S2 cells. Importantly, Arf1 inhibition also inhibited Fz delivery to the apical junctional regions in vivo , where it must localize to participate in PCP establishment. We propose a model whereby Arf1/AP-1 are involved in the specific transport of the PCP-core factor Fz, and most likely also Vang and Fmi, to the PM during PCP establishment, a process required for enrichment of these proteins in polarized complexes. Recently, it was shown in a mammalian non-polarized culture system that Vangl2 trafficking out of the Golgi depends on Arfaptin and the AP-1 complex [22] , which is consistent with our data and supports the evolutionary conserved task for these proteins in promoting PCP-core component localization. Arf1 can also act through the COPI complex (reviewed in ref. 42 ), and, for example, in flies, at the cis-Golgi, Arf1 together with its guanine nucleotide exchange factor/GEF Gartenzwerg regulate COPI retrograde transport [52] . We thus also tried to test this possibility. However, the dsRNA-based KD in vivo of all COPI complex components is cell lethal and thus not informative in this context. Similarly, in cell culture COPI KD, depending on the level, was either too toxic or failed to show an effect on Fz trafficking. As such, although we cannot completely exclude that COPI is also involved in the process, we trust that the comparable results of Arf1 and AP-1 indicate that Arf1 acts at least in part on AP-1 in PCP trafficking. Several studies have identified genes that affect localized actin hair formation in Drosophila wing cells. Interestingly, apart from the PCP-core components, these usually fall into two cellular machinery categories: actin polymerization-related proteins and trafficking-related proteins (reviewed in ref. 3 ). Importantly, both sets of factors have been linked to each other in diverse cellular environments, including carrier formation at the Golgi [53] , yeast budding [54] , formation of phagocytic cups [55] , [56] or lamellipodia formation in migrating cells [57] . Silencing of Arf1, Rab11, PI4KIIIβ and AP-1 leads to defects in actin-based hair formation in wing cells, notably leading to the formation of mch. Using Drosophila S2 cells, Humphreys et al. [58] described that Arf1 is found not only in the Golgi but also at actin-rich cell edges, and that it is essential for lamellipodium biogenesis. In vertebrates, Arf1 is also required for actin polymerization, for example, in neuronal tissues during plasticity Arf1 regulates Arp2/3 through PICK1 (ref. 59 ). Based on these data, a direct/parallel involvement of the Arf1 protein network is likely during hair formation, and indeed we observe an enrichment of these proteins in the growing actin hairs ( Fig. 8 and ref. 41 ; see also model in Fig. 10 ). Thus, in summary, our data on Arf1/AP-1 and its network suggest that it functions repeatedly in different PCP establishment processes, ranging from the initial PCP-core component localization to later restricting the foci of actin polymerization. 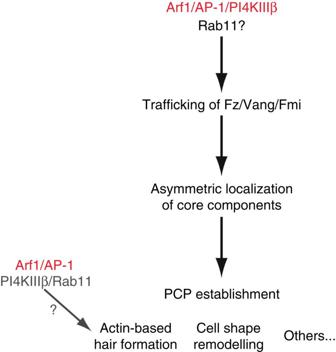Figure 10: Working model for AP-1 and Arf1 function in PCP. See main text for details. Figure 10: Working model for AP-1 and Arf1 function in PCP. See main text for details. Full size image Fly stocks Flies were raised on standard medium and maintained at 25 °C, unless otherwise indicated. GAL4/UAS system [60] was used for gene expression and RNAi studies. The Gal4 expression drivers were as follows: en-GAL4, nub-GAL4 , sev-Gal4 and pnr-Gal4 . In addition, to avoid lethality of Arf1 T31N expressing flies, we used the eye-specific sev-promoter- Gal4 driver, sep-Gal4 , to express the transgene in the eye. In addition, the following lines were used: Arf1 Q71L and Arf1 T31N (a gift from S.F. Onel), Arf1-WT (a gift from T. Harrys), AP47-VFP and AP-1 mutant AP47 SHE11 (gift from R. Le Borgne) , fwd Z0453 (gift from J. Brill), fz p21 (Bloomington Stock Center), fz RNAi (VDRC v43075), mwh RNAi (VDRC v45265), gish RNAi ref. 41 , Rab11 Q70L (Bloomington Stock Center) and fwd RNAi (Bloomington Stock Center and VDRC v110159). Other Drosophila lines were developed in this study as indicated below. Zebrafish husbandry Zebrafish husbandry were conducted in accordance to standard protocols and adhered to Canadian Council of Animal Care guidelines. In situ hybridization was conducted according to (Hayes et al. [31] ) using myoD and krox20 antisense RNA probes generated by in vitro transcription (DIG RNA Labeling Kit, Roche). Transgenic flies, plasmids and expression constructs DmrD4-Fz into pAc-GFP vector : The signal sequence, four copies of the dimerization domain ( DmrD) and a furin cleveage site were cloned by PCR into the pAc5-STABLE-1-puro (a gift from J. Sutherland) using the oligos forward 5′-GGGGTACCATGGCTACAGGCTCC-3′ and reverse 5′-GGGGTACCCTCTCTCTTCTGACGGTTTC-3′ and Clontech vector prHom-Sec1 as a template. KpnI restriction site was used to introduce the 4xDmrD sequences. Drosophila Frizzled coding region without the signal sequence and with a myc tag inserted after the CRD domain was cloned by PCR from our previous vector [48] with the oligos forward 5′-CCGGAATTCTACGATCAGAGCCCCCTC-3′ and reverse 5′-CCGGAATTCGACGTACGCCTGCGCC-3′ and clone in the EcoRI site to generate the final pAc-DmrD4-Fz-EGFP. DmrD4-Fz-GFP into pUASt vector The DmrD4-Fz-EGFP coding sequence was then subcloned into the Drosophila expression vector pUASt using the following primers: forward 5′-ATAAGAATGCGGCCGCATGGCTACAGGCTCCCGG-3′, and reverse 5′-ATAAGAATGCGGCCGCTCAGTACAGCTCGTCCAT-3′. PI4KIIIβ into pUASt vector and pAc 5-1 To generate UAS-GFP-PI4KIIIβ transgenic flies, GFP-PI4KIIIβ sequence was subcloned by PCR into pUASt vector and pAc 5.1. We used the pCasperhs83-GFP-Fwd vector (gift from J. Brill) as a template and amplified GFP-forward sequence with the following primers: 5′-GCGCGGCCGCCATGGTGAGCAAGGGCGAGG-3′ and 5′-CGTCTAGAGTCACAATATGCCATTAGTGTAGTATTG-3′. hArf1 into pAc 5.1-Flag-Cherry We first generated a pAc 5.1 vector containing Flag-Cherry using the KpnI and EcoRI restriction sites. For that we used pAc5-STABLE-2 (a gift from J. Sutherland) as template and then PCR amplified the Flag-Cherry sequence with the following primers: forward 5′-ACGGTACCATGGACTACAAAGACGATGAC-3′ and reverse 5′-ACGAATTCTTTATACAGCTCGTCC-3′. Once we had the pAc 5.1-Flag-Cherry, we cloned the WT version of the human Arf1 in the KpnI site using as a template for the PCR the vector pARF1-CFP (Addgene ID: 11381) with the following primers: forward 5′-ACGGTACCATGGGGAACATCTTCG-3′ and reverse 5′-ACGGTACCCTTCTGGTTCCGGAGC-3′. Plasmids and microinjections in zebrafish studies All human Arf1 isoforms (hArf1-WT, hArf1 Q71L ) were PCR amplified (forward primer: 5′-GGGGACAAGTTTGTACAAAAAAGCAGGCTTCGCCACCATGGGGAACATCTTCGCCAACCT-3′ and reverse primer: 5′-GGGGACCACTTTGTACAAGAAAGCTGGGTGCTTCTGGTTCCGGAGCTGATT-3′) from pECFP-N1 vectors and cloned into pCS2Dest2 (ref. 61 ) using Gateway Technology (Invitrogen). mRNA for microinjections was synthesized in vitro using mMESSAGE mMACHINE (Ambion) and injected into one-cell-stage WT embryos in the following amounts: hArf1-WT-GFP and hArf1 Q71L− GFP (120, 75, 45, 30, 20, 15 and 10 pg), and membrane-localized monomeric red fluorescent protein (10 pg). Immunostaining and histology For analysis of wing trichomes, adult wings were removed, incubated in wash buffer (PBS and 0.1% Triton X-100 (PBT)) and mounted on a slide in 80% glycerol in PBS. Eye sections were prepared as described before [62] . Eyes were sectioned near the equatorial region and only ommatidia with the correct photoreceptor number were scored for PCP defects. Phenotypes in the eye were scored for rotation, chirality and loss/gain of photoreceptors of individual ommatidia. Adult wings and eye sections were imaged at room temperature on a microscope (Axioplan; Carl Zeiss). Images were acquired with a camera (Zeiss AxioCam Color type 412–312; Carl Zeiss) and AxioCam software. For analysis of pupal wings, prepupae (white pupae) were collected and staged at 25 °C for 30–32 h for pupal wings. Wings were dissected and fixed in PBS, 4% formaldehyde and 0.1% Triton X-100 for 45 min. Tissues were washed twice in PBT and incubated in PBT 2% BSA for 30–45 min. Primary antibodies were incubated overnight at 4 °C. Samples were washed five times in PBT and incubated for 1 h in fluorescent secondary antibodies diluted in PBT. Five additional washes in PBT were performed before mounting on slides with Vectashield (Vector Laboratories). Pupal wing images were acquired at room temperature using a confocal microscope ( × 40 ∼ oil immersion, 1.4 numerical aperture; SP5 DMI; Leica) with LAS AF (Leica) software. Images were processed with ImageJ (National Institutes of Health) and Photoshop (CS4; Adobe). Antibodies Primary antibodies were as follows: rabbit anti-Fz (1:300, gift from D. Strutt), rat anti-Stbm (1:1,000, gift from D. Strutt), anti-GFP (1:1,000, Invitrogen, cat. no. MA5-15349), mouse anti-myc (1:500, Santa Cruz, cat. no. sc-40[9E10]), rat anti-DE-cadherin (1:20, developmental studies hybridoma bank (DSHB) non-commercial), mouse anti-Fmi (1:10, DSHB), anti-FasIII (1:10, DSHB), LqfR (1:100; gift from J. Fischer), Hrs (1:1,000; gift from H. Bellen), Rab5 (1:1,000, Abcam, cat. no. ab31261) and anti-AP-1γ (1:100 gift from R. Le Borgne). Rhodamine–phalloidin (1:500; gift from C. Iomini). Fluorescent secondary antibodies were obtained from Jackson Laboratories and Invitrogen (Alexa 568). DmrD4 studies in cell culture and in vivo See the Supplementary Information for a detailed description associated with these studies ( Supplementary Fig. 5 ). Localization analysis in S2 cells S2 cells were cultured at 25 °C in Schneiders media (Gibco) supplemented with 10% heat-inactivated fetal bovine serum and penicillin/streptomycin. S2 cells were transfected with the desired combination of plasmids (hArf1-Cherry, GFP-PI4KIIIβ and HA-Rab11) using Effectene transfection reagent (Qiagen). Then cells were cultured in regular media for 48 h before plating them in low concentration on concanavalin A-coated coverslips for low spreading. Cells were fixed 30–60 min after seeding with 4% PFA, washed three times with PBS and processed for inmunofluorescence. After washes, coverslips were mounted with Vectashield (Vector Laboratories). Cell images were acquired using a fluorescence microscope ( × 63 ∼ oil immersion, 0.8 numerical aperture; DM5500B; Leica) with LAS AF (Leica) software. Images were processed with ImageJ (National Institutes of Health). Fluorescence image quantifications Polarity vector for individual cells were calculated with the software packing_analyser_V2 as described [11] based on anti-Fmi staining. The software calculated both angles (relative to the P–D axis for example) and strength of polarization (nematic order). Nematic order is calculated as the strength (extent) of polarization and angle is calculated as the direction of polarization within a cell [11] ). Both measurements are based on the staining intensity of core PCP factors around the cell membrane. The resulting polarity ‘angle lines’ were then processed using the MATLAB software [63] for rosette diagram presentations. χ 2 -Test was used for statistical analyses. Cellular packing was also calculated using the software packing_analyser_V2 (ref. 11 ). Fluorescence intensity quatification for Fmi, Fz, Vang, DE-Cad and FasIII was done with ImageJ [64] selecting the different cell junctions (close to 90 or 0 degrees) with the Draw line tool and calculating the grey intensity value. Junctional planes of the Z-stack for Fmi, Fz, Vang and DE-cadherin and a single subapical plane for FasIII were used for quantifications. Confocal imaging for zebrafish Live embryos labelled with membrane red fluorescent protein were anaesthetized and immobilized onto glass coverslips in 1% agarose, embryos were dorsally mounted to acquire Z-stack images of the dorsal ectoderm and notochord [65] . Images were taken using a Zeiss LSM 710 microscope and processed using ImageJ software. For dorsal ectoderm LWR analysis, the LWRs of cells were obtained by imaging a single plane of dorsal ectoderm cells at 90% epiboly. Ratios were then calculated by dividing the long axis of each cell by its short axis using Microsoft Excel 2010 software. Statistical analyses Comparisons between samples for number of mch per wing, polarity vector length, cell area and mean fluorescence intensity were performed with the t -test. Polarity vector distributions were compared using the χ 2 -test. For zebrafish data studies, all statistical analyses were performed using the two-tailed paired t -test. How to cite this article: Carvajal-Gonzalez, J. M. et al. The clathrin adaptor AP-1 complex and Arf1 regulate planar cell polarity in vivo . Nat. Commun. 6:6751 doi: 10.1038/ncomms7751 (2015).